Voltage tunability of single-spin states in a quantum dot Single spins in the solid state offer a unique opportunity to store and manipulate quantum information, and to perform quantum-enhanced sensing of local fields and charges. Optical control of these systems using techniques developed in atomic physics has yet to exploit all the advantages of the solid state. Here we demonstrate voltage tunability of the spin energy-levels in a single quantum dot by modifying how spins sense magnetic field. We find that the in-plane g -factor varies discontinuously for electrons, as more holes are loaded onto the dot. In contrast, the in-plane hole g -factor varies continuously. The device can change the sign of the in-plane g -factor of a single hole, at which point an avoided crossing is observed in the two spin eigenstates. This is exactly what is required for universal control of a single spin with a single electrical gate. The spin of charges in quantum dots (QDs) has long been considered a suitable qubit for quantum operations [1] . The three-dimensional confinement offered by a single semiconductor QD reduces many decoherence mechanisms, allowing impressively long coherence times to be observed in coherent population trapping [2] or using spin-echo techniques [3] , [4] . In the latter, control of the spins was achieved with resonant, ultrafast optical pulses. An alternative mechanism for controlling single spins is for an electric field to vary their coupling to a fixed magnetic field ( B ), described by the g -tensor ( g ) [5] . This method allows multiple closely spaced spin qubits to be individually addressed via nano-electrodes, without resonant lasers or localized magnetic fields. Critical to this concept is the ability to change the sign of one component of the g -tensor [5] , [6] . Then through careful alignment of the magnetic field direction it is possible to switch between two electric fields where the precession directions of the spin (given by g.B ) are orthogonal on the Bloch sphere. In such a system, ‘universal’ control can map any point on the Bloch sphere onto any other point. Although experimental studies have been made of the g -tensor in QDs [7] , [8] , [9] , [10] , [11] , [12] , the change of sign of one component with electrical field has yet to reported. Early work used semiconductor quantum wells to electronically tune the g -tensor of multiple spins by shifting their carrier wavefunctions into areas of different material composition [13] . Extending this work to single charges trapped in zero-dimensional structures has not been straightforward as the carriers tunnel out of the structure when electric field is applied. One approach was demonstrated using electronically coupled pairs of QDs [14] . Carriers displayed the g -tensor of the material in which they were located, so when a voltage was applied to localize the charge in one dot, the g -factor measured was that of the indium-rich QD. However, when the wavefunction was delocalized between the dots, there was a much greater spatial overlap with aluminium arsenide semiconductor in the barrier, and a change in g was observed. Recently, experiments showed that vertical electric fields can change the g -factor relevant for out-of-plane magnetic fields ( g ┴ ) [9] in dots that are engineered to have increased height and reduced indium composition. The in-plane g -factor of an s -shell hole ( ) was also modified by vertical electric field [10] over a modest field range of 20 kV cm −1 . However, both of these measurements were made in the photo-current regime, where carriers rapidly tunnel from the dot greatly limiting the spin lifetime. Conversely, an in-plane electric field can change the g -tensor, but there the tunnelling problem is even more severe [11] , [12] . We solve these problems by locating single dots in the centre of a p - i - n diode where barriers that hinder tunnelling allow us to apply electric fields, F , up to −500 kV cm −1 , while still observing photoluminescence [15] . We study changes in the g -tensor as a function of electric field and show that a high degree of control can be achieved for both electrons and holes. We observe that continuous variation in the g -factor of holes in a parallel magnetic field can be obtained. Different behaviour is observed depending on whether the hole is in the s - or p -shell. When has a low value at zero electric field these devices are capable of tuning it through an avoided crossing at finite field, and changing its sign, without carriers escaping. Charged exciton transitions in magnetic and electric field When the magnetic field is orthogonal to the plane of the sample (Faraday geometry, B ┴ ), we see that the g -factors are barely affected by electric field (see Supplementary Fig. S1 and Supplementary Note 1 ). However, when the magnetic field is aligned in the plane of the sample (Voigt geometry, B || ), strikingly different behaviour is observed. The separate in-plane g -factors of s -shell electrons ( ) and holes ( ) may be determined from the decay energies of the positively ( X + ) and negatively ( X − ) charged excitons. The magnetic field splits both the upper ( ) and lower states ( ) of X − , where μ B is the Bohr Magneton. Four transitions ( E 1 – E 4 ) are observed as shown in Fig. 1a . The highest and lowest energy transitions of this quadruplet ( E 1 and E 4 ) emit photons with electric field orthogonal to B and the intermediate transitions ( E 2 and E 3 ) parallel to B . Fitting the energies of each transition resulting from the X − state, one can determine and using and . Similar arguments can be made to determine and from the X + transitions. There is not enough information in this measurement alone to determine the sign of these g -factors. However, for nearly all dots, we see an increase in the fine-structure splitting of the neutral exciton state with magnetic field, which is a signature that both have the same sign [16] , which we take to be negative [14] , [17] . 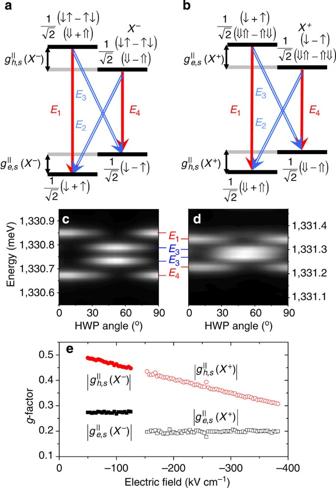Figure 1: Electric field tuning ofs-shell electron and holeg-factors. (a,b) The energy levels of the negatively and positively charged excitons (X−andX+, respectively) in a Voigt-geometry magnetic field is showed. TransitionsE1andE4(red) result in linearly polarized emission orthogonal to the magnetic field, andE2andE3(blue) are parallel to the magnetic field. (c,d) Polarization-dependent spectra from theX−at −78.5 kV cm−1andX+at −385.7 kV cm−1, respectively, at a field of 4T, as a half-wave plate (HWP) is rotated. (e) The extracteds-shell electrong-factor,, ands-shell holeg-factor,, as a function of electric field is showed. Figure 1: Electric field tuning of s -shell electron and hole g -factors. ( a , b ) The energy levels of the negatively and positively charged excitons ( X − and X + , respectively) in a Voigt-geometry magnetic field is showed. Transitions E 1 and E 4 (red) result in linearly polarized emission orthogonal to the magnetic field, and E 2 and E 3 (blue) are parallel to the magnetic field. ( c , d ) Polarization-dependent spectra from the X − at −78.5 kV cm −1 and X + at −385.7 kV cm −1 , respectively, at a field of 4T, as a half-wave plate (HWP) is rotated. ( e ) The extracted s -shell electron g -factor, , and s -shell hole g -factor, , as a function of electric field is showed. Full size image appears to be constant for a given exciton complex, but on switching between the X + and X − transitions an abrupt step is always observed. The reason for this is that is determined by the initial state (when there are two holes also present in the dot). These holes are better confined than the electron and provide a coulomb attraction that reduces the extent of the electron wavefunction, pushing closer to +2(ref. 18 ). However, when no holes are present is determined from the final state of the X − transition. For the sample of 15 dots studied and , where the numbers quoted are the mean±s.d. In contrast to the behaviour of the electron, varies linearly with electric field for both X + and X − in Fig. 1e . We estimate that the discontinuity in on switching between X + and X − is on average an order of magnitude smaller than the similar effect for , as expected, given the greater spatial extent of the electron wavefunction. There is remarkable homogeneity in the rate at which can be tuned with electric field for different dots, cm kV −1 , where at zero electric field is 0.469±0.110. The scatter in the value of at F =0 is greater than the comparable value for the electron, as this is affected more strongly by variations in dot height and lateral size [18] . The rate ξ compares well with the recent publication of Godden et al . [10] , which determines from the energy splitting of the X − in a time-resolved photo-current measurement. This paper reports a linear variation in at a rate of 3.5 × 10 −4 cm kV −1 over a range of only 20 kV cm −1 . The rate of shift is also of the same order of magnitude as that predicted theoretically, for dots of greater height and uniform composition [6] . It will be interesting to see whether further theoretical work can fully explain the variations in the g -tensor we observe. Minimizing the g -factor of the s -shell hole With the range of fields accessible in these samples, any dot with 0.285 at F =0 can be tuned to a minimum at some field, F 0 . We now discuss data from a dot with =0.174 at F =0. This same QD also displays a minimum in the fine-structure splitting of the neutral exciton of 1.8 μeV at −57.1 kV cm −1 . We find that cm kV −1 , and thus we are able to tune the hole eigenstate splitting Δ= towards a minimum value at an electric field of F 0 =−225.0 kV cm −1 . For fields above F 0 (such as shown in Fig. 2a ), we observe that the sign of is the same as for all other dots in the ensemble. For electric fields below F 0 (such as in Fig. 2e ), has the opposite sign, which manifests itself as a clear difference in the orientation angle at which the largest difference in transition energies is observed. 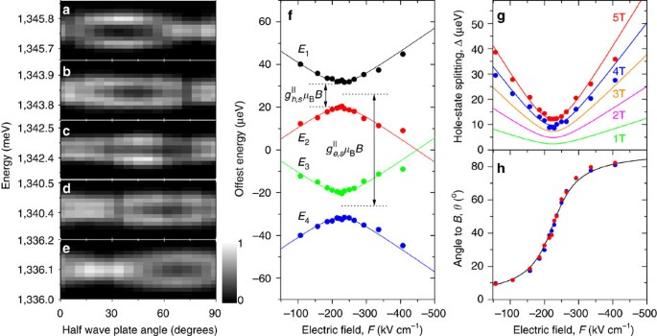Figure 2: Changing the sign of the Voigt-geometrys-shell holeg-factor with electric field. Polarized spectra of the positively charged exciton,X+, for an in-plane magnetic field of 5T and electric fields of (a) −107.1 kV cm−1, (b) −185.7 kV cm−1, (c) −221.4 kV cm−1, (d) −264.3 kV cm−1and (e) −335.7 kV cm−1. (f) The energies of the four transitions of theX+offset by their mean value at each electric field is showed. (g) The magnitude of the holeg-factor,, and the (h) orientation (θ) of the states relative to the magnetic field. Bothg,hshow fits for 1–5T based on equations (1) and (2). Figure 2f plots the X + transition energies as a function of electric field, F , to clearly show the form of the anti-crossing in the hole states (the mean value of all four transition energies has been subtracted for clarity, to remove the Stark shift). The minimum hole-state splitting corresponds to 0.042, but we stress that on either side of this minimum value, the has different sign. Figure 2: Changing the sign of the Voigt-geometry s -shell hole g -factor with electric field. Polarized spectra of the positively charged exciton, X + , for an in-plane magnetic field of 5T and electric fields of ( a ) −107.1 kV cm −1 , ( b ) −185.7 kV cm −1 , ( c ) −221.4 kV cm −1 , ( d ) −264.3 kV cm −1 and ( e ) −335.7 kV cm −1 . ( f ) The energies of the four transitions of the X + offset by their mean value at each electric field is showed. ( g ) The magnitude of the hole g -factor, , and the ( h ) orientation ( θ ) of the states relative to the magnetic field. Both g , h show fits for 1–5T based on equations (1) and (2). Full size image The behaviour of Δ is reminiscent of the anti-crossing in neutral exciton states that has been observed with electric field [15] , [19] , [20] , however, in this case the states that are coupled together contain only a single hole. Indeed, in the analysis of Plumhof et al . [21] who studied the anti-crossing of the neutral exciton states under externally applied strain, it was the hole wavefunction that dominated the orientation of the eigenstates relative to the laboratory ( θ ) and anti-crossing of the eigenenergies. As with the neutral exciton, we fit the avoided crossing with a coupling parameter , where the splitting between the hole states varies linearly away from F 0 at a rate ξμ B B || . In Fig. 2g , we show data summarising the behaviour of the two hole eigenstates at 4T (the lowest field at which we can spectrally resolve all four transitions) and 5T (the highest field available with our magnet) fitted with this model. We observe that the magnitude of the anti-crossing in energy appears to scale linearly with B || , thus is constant, at least in the range of fields we can probe. The resulting variation of θ with F is the same for both magnetic fields ( Fig. 2h ), in accordance with equations (1) and (2). It will be interesting to further probe the behaviour of this effect in higher magnetic fields. g -factor of the p -shell hole Finally, we study the decay of the positively changed biexciton, XX + , which consists of a filled s -shell and a excess p -shell hole. These transitions are observed on the low-energy side of the X + transition [22] , [23] . We determine the g -factors of the p -shell hole which, to our knowledge, has not been possible before (although the Voigt-geometry electron p -shell g -factor has been probed [24] ). We find that in the Faraday geometry, there is no variation in the p -shell hole g -factor as a function of electric field. In a Voigt geometry, the brightest radiative decays from XX + involve recombination of an s -shell electron and hole. The resulting photons are linearly polarized as shown in Fig. 3a (blue and red arrows have orthogonal linear polarization), with the initial state XX + split by , where is the Voigt p -shell hole g -factor. However, the final states can either have spin S =1/2 or 5/2: their splittings are partly determined by the electron-hole exchange between the s -shell electron and p -shell hole, which has not been well studied. Empirically, we see that the spin splitting of the S =1/2 final state is below the system resolution at B || =0, but increases with magnetic field. In contrast, the S =5/2 final state has a spin splitting of several hundred μeV at B || =0 but is reduced with B || . Nevertheless, it is possible to measure the initial-state splitting XX + using either the S =1/2 or S =5/2 final state quadruplets, and thus infer . When this is done, both quadruplets lead to the same value of ( Fig. 3e ), as expected. We find that has a greater magnitude than and varies non-linearly with electric field. The greater extent of the p -shell hole wavefunction outside the dot is likely to bring closer to the value determined by the wetting layer and surrounding Gallium arsenide (GaAs). 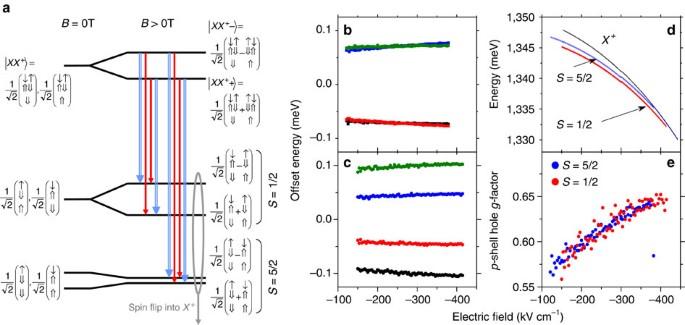Figure 3: Determination of Voigt-geometryp-shell holeg-factor. (a) The allowed transitions for recombination of ans-shell electron-hole pair of the positively charge biexciton,XX+, is showed. Red and blue arrows indicate photon emission with opposite linear polarization. (b) The energies of the quadruplet withS=5/2 final state, offset by their mean at 4T, and (c) the energies of the quadruplet withS=1/2 final state, offset by their mean at 4T, as a function of electric field. (d) The absolute energy of the transitions shown inaversus electric field, at 4T. Fromb,c, we independently extract the magnitude of thep-shell holeg-factor (e) for theS=1/2 (red) andS=5/2 (blue) transitions. Figure 3: Determination of Voigt-geometry p -shell hole g -factor. ( a ) The allowed transitions for recombination of an s -shell electron-hole pair of the positively charge biexciton, XX + , is showed. Red and blue arrows indicate photon emission with opposite linear polarization. ( b ) The energies of the quadruplet with S =5/2 final state, offset by their mean at 4T, and ( c ) the energies of the quadruplet with S =1/2 final state, offset by their mean at 4T, as a function of electric field. ( d ) The absolute energy of the transitions shown in a versus electric field, at 4T. From b , c , we independently extract the magnitude of the p -shell hole g -factor ( e ) for the S =1/2 (red) and S =5/2 (blue) transitions. Full size image Several proposals exist for universal control of a single spin in a QD [1] , [5] , [6] , [25] . The ability of the device reported here to change the sign of , combined with the reduced hole–hyperfine interaction and greater hole-spin lifetime open up the possibility of all-electrical 4 π manipulation of the hole spin. Alternatively, controlled phase shifts may be achieved on a qubit encoded on the spin of the electron by addition of two holes for a predetermined time, which could be achieved by controlled charging. The timescale of any electrical control sequence is limited by the resistance and capacitance of the diode to tens of picoseconds [26] , which is significantly greater than that achieved with coherent optical pulses. However, the ability to achieve full Bloch-sphere control with only a single electrical gate is a promising avenue of investigation. Such a device could find applications in a spin-based quantum memory [27] , spin-echo techniques [3] , [4] , spin-based quantum computing [1] , [28] and generation of photonic cluster-states [29] . Sample design The sample consists of a single layer of self-assembled QDs grown in the centre of a 10-nm wide GaAs quantum well, clad with a 75% AlGaAs superlattice, which suppresses the tunnelling of carriers. These dots are grown in a single deposition of InAs at a substrate temperature of 470 °C and with a transition to self-assembled 3D growth at 60 s. The resulting dots are 2–3 nm in height, and are capped in 5 nm of GaAs at 470 °C before raising the substrate temperature for growth of the superlattice. p - and n -doping regions are arranged symmetrically above and below the QD layer, with a total intrinsic region thickness of 140 nm. The diode is encased in a weak planar microcavity, with micron-sized apertures in a metallic layer on the surface to allow optical addressing of single dots. Experimental arrangement The sample is mounted inside the bore of a superconducting magnet applying fields of up to 5T. When the sample growth direction is aligned with the magnetic field, a single on-axis microscope objective is used to excite and collect the emission from the sample. When the magnetic field is in the plane of the sample (Voigt geometry), an additional 45° mirror is mounted to allow optical access to the sample. Photoluminescence is excited from the sample with a continuous wave 850 nm laser diode, and passed through a rotatable half-wave plate and polariser before detection. For the data in Fig. 2 , spectral measurements confirm that the sample was orientated within 0.1° of the magnetic field direction. How to cite this article: Bennett, A. J. et al . Voltage tunability of single-spin states in a quantum dot. Nat. Commun. 4:1522 doi: 10.1038/ncomms2519 (2013).